Three-dimensional shape transformations of hydrogel sheets induced by small-scale modulation of internal stresses Although Nature has always been a common source of inspiration in the development of artificial materials, only recently has the ability of man-made materials to produce complex three-dimensional (3D) structures from two-dimensional sheets been explored. Here we present a new approach to the self-shaping of soft matter that mimics fibrous plant tissues by exploiting small-scale variations in the internal stresses to form three-dimensional morphologies. We design single-layer hydrogel sheets with chemically distinct, fibre-like regions that exhibit differential shrinkage and elastic moduli under the application of external stimulus. Using a planar-to-helical three-dimensional shape transformation as an example, we explore the relation between the internal architecture of the sheets and their transition to cylindrical and conical helices with specific structural characteristics. The ability to engineer multiple three-dimensional shape transformations determined by small-scale patterns in a hydrogel sheet represents a promising step in the development of programmable soft matter. There is a growing interest in mechanically active, self-shaping materials that undergo a desired, prescribed three-dimensional (3D) shape transformations, on demand, under the action of an external trigger [1] , [2] , [3] , [4] . One of the approaches to the design of such materials utilizes the generation of non-uniform internal stresses [5] , [6] , [7] , [8] , [9] , [10] , [11] , [12] . In the past decade, bending and folding of soft elastic sheets have been achieved by inducing gradients in swelling across the sheet thickness [11] . Recently, in-plane differential swelling was introduced as a new concept of 3D shape transformations of thin gel sheets [5] , [10] . A non-uniform swelling field was prescribed to the sheet by modulating the concentration and the crosslinking density of the temperature-responsive polymer. This strategy paved the way for shape transformations that were not attainable in earlier works, however, the method of sheet construction required rigorous fine-tuning of the continuous, smooth swelling fields and was difficult to implement. More importantly, a single stable shape change was preprogrammed in the material and subsequently, activated by applying a particular stimulus (heating). It turns out that nature has found a remarkable way to use sharp lateral modulation in swelling for the self-shaping of fibrous plant organs [13] , [14] , [15] . Fibrous tissue consists of long, narrow and relatively rigid fibres embedded in a soft, pliant matrix. Fibres may differ from the matrix not only in their rigidity, but also in their expansion or swelling properties and may orient differently in the different layers of the matrix [15] , [16] . In response to changes in ambient humidity, shape transformations of plant organs are governed by differences in the swelling of different components of the fibrous tissue. Being inspired by the mechanically active nature of plant organs, we developed a new self-shaping approach that mimics morphological transformations of fibrous tissues, but utilizes a single-layer material, made of stripes with alternating chemical compositions. As an example of shape transitions, we focused first, on helical structures that are frequently encountered in fibrous organs of plants. Valves of pods of many vetches and awns of wild oats, Aaenafatua L. , or feather grass, Stippa , to name a few systems, form helices under desiccation [13] , [14] . In these examples, as well as in man-made systems [16] , [17] , [18] , [19] , [20] , planar-to-helical transformations and bending, in general, are achieved for bimorph sheets with different properties of the top and the bottom surfaces, which cause the generation of a uniaxial or a biaxial spontaneous curvature. In the present work, the new shaping mechanism was governed by small-scale, sharp modulations in swelling and mechanical properties of fiber-like structural components of the single-layer material. We designed a hydrogel sheet with periodic stripes of different compositions, passing at an oblique angle, θ , with respect to the long axis of the sheet. The critical design rule was such that an external stimulus induces a large difference in the swelling/shrinkage ratios and elastic moduli of the two types of stripes. The transformation of the planar sheet into a helix was driven solely by the reduction in stretching energy, and it yielded cylindrical helices with equally probable right- and left-handedness (an optional control over helix chirality was achieved by inducing a difference in hydrogel composition across the sheet thickness). In contrast with bending- or twist-mediated transitions reported by other groups [16] , [17] , [18] , [19] , [20] , the shape transformations were mediated solely by in-plane forces and did not require a difference in structure or composition across the thickness of the sheet. The proposed mechanism was validated by the generation of cylindrical and conical helical structures with prescribed structural characteristics, by transitions between the two helical states with a different number of turns, and by multiple, distinct and stable shapes activated by different external stimuli. The method was robust and because of the small-scale chemically distinct structural units, it was suitable for the construction of multi-component, reconfigurable ‘digital materials’. Shape transformations of hydrogel sheets A sheet of poly( N -isopropylacrylamide (PNIPAm)) hydrogel (a primary gel, PG) was swollen with an aqueous solution of 2-acrylamido-2-methylpropane sulphonic acid (AMPS), N , N ′-methylene- bis -acrylamide (MBAA) and a 2,2'-azo- bis -(2-methylpropionamidine), and subjected to ultraviolet light irradiation through a photomask ( Fig. 1a and Supplementary Fig. S1 ). Photopolymerization generated an interpenetrating network of PNIPAm/poly(AMPS) (PNIPAm/PAMPS) (a binary gel, BG) in the light-exposed regions of the sheet. The stripes of PG and BG are shown with light-blue and dark-blue colours, respectively ( Fig. 1a ). The stripes were aligned along the x -direction, while the y -direction was transverse to the stripes and the z -direction was along the sheet thickness. The combination of PNIPAm and PNIPAm/PAMPS stripes enabled a strong modulation of the properties of PG and BG stripes, owing to the heat- or ionic strength-mediated dehydration of PNIPAm and the retention of water by PAMPS [21] , [22] , [23] . In deionized water heated to 45 °C, above the temperature of dehydration of PNIPAm, and in an aqueous NaCl solution, a patterned sheet underwent a reversible transition to a helix ( Fig. 1b , Supplementary Figs. S2 and S3 , and Supplementary Movies S1 and S2). 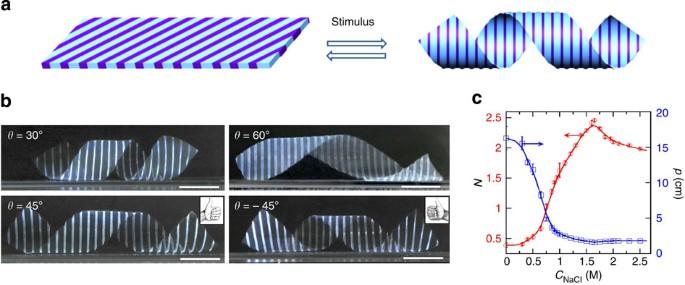Figure 1: Formation of helical structures. (a) Left: A planar sheet of the composite gel patterned with 1 mm-wide stripes of PNIPAm gel (PG) and PNIPAm/PAMPS gel (BG) passing at an angleθto the long axis of the sheet. The dark and light-blue colours correspond to the stripes of PG and BG, respectively. Right: A helix formed by the composite gel sheet under the action of external stimulus. (b) Images of the helices generated after 24 h incubation of the gel sheets with the initial thickness in a 1 M NaCl solution. The hand symbols indicate the handedness of the helix. The labels on the images show the value of angleθ. The thickness of the sheett0=0.44 mm. The radius of the helix was ~0.5 cm. Scale bar, 1 cm. (c) Variation in pitch,p, and the number of turns,N, of the left-handed helix (θ=45°), plotted as a function of the concentration of NaCl solution. Following photoirradiation, the top surface of the hydrogel was exposed for 5 min to the ambient air.t0=0.44 mm. The error bars represent s.d. values calculated from three measurements. Figure 1: Formation of helical structures. ( a ) Left: A planar sheet of the composite gel patterned with 1 mm-wide stripes of PNIPAm gel (PG) and PNIPAm/PAMPS gel (BG) passing at an angle θ to the long axis of the sheet. The dark and light-blue colours correspond to the stripes of PG and BG, respectively. Right: A helix formed by the composite gel sheet under the action of external stimulus. ( b ) Images of the helices generated after 24 h incubation of the gel sheets with the initial thickness in a 1 M NaCl solution. The hand symbols indicate the handedness of the helix. The labels on the images show the value of angle θ . The thickness of the sheet t 0 =0.44 mm. The radius of the helix was ~0.5 cm. Scale bar, 1 cm. ( c ) Variation in pitch, p , and the number of turns, N , of the left-handed helix ( θ =45°), plotted as a function of the concentration of NaCl solution. Following photoirradiation, the top surface of the hydrogel was exposed for 5 min to the ambient air. t 0 =0.44 mm. The error bars represent s.d. values calculated from three measurements. Full size image The morphology of the helix changed with the angle θ ( Fig. 1b , Supplementary Fig. S4 , and Supplementary Table S1 ). For 30≤ θ ≤60°, more compact helices formed at a lower value of θ . For a particular angle θ , left-handed and right-handed helices formed with equal probability ( Supplementary Fig. S5 ). For such sheets, an optional control over helix handedness was achieved by using a mask with θ =45° and θ =−45°, respectively. In addition, for θ =45°, an optional control over helix chirality could be achieved by quenching polymerization of PAMPS at one of the sheet surfaces [24] ( Supplementary Fig. S6 ; Supplementary Methods ). Subsequently to that, in an aqueous medium, the surface deprived of PAMPS surface underwent a weaker swelling than the other surface and formed the inner surface of the helix. For a particular design of the hydrogel sheet, the structural characteristics of the helix such as the number of turns, N , and the pitch, p , were controlled by varying the concentration of NaCl solution, C NaCl ( Fig. 1c and Supplementary Fig. S7 ). The most compact helix was formed at C NaCl =1.7 M, whereas in less and more concentrated NaCl solutions the helical structure was more relaxed. Properties of structural elements of the composite gel sheet To explore the mechanism of helix formation, we examined the properties of individual PG and BG gels in solutions with a varying C NaCl . 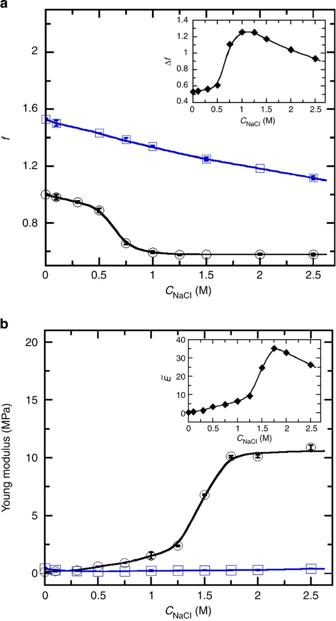Figure 2: Variation in properties of the individual PG and BG components of the patterned gel sheet. (a) Relative change in the linear dimensions,f, of PG (○) and BG (□), plotted as a function ofCNaCl. (b) Variation in the Young’s moduli of PG (○) and BG (□), plotted versusCNaCl. The error bars represent s.d. calculated from three measurements. Insets inaandbshow the variation in the normalized difference in dimensions of PG and BG,Δf, and the ratio of Young’s moduli,, respectively. Figure 2a shows the relative change in the dimensions of PG and BG, f = d / d 0 , where d and d 0 are the diameters of the corresponding gel disks in NaCl solution and immediately after the synthesis, respectively. The dimensions of PG strongly decreased at 0.5≤ C NaCl ≤1.0 M, owing to PNIPAm dehydration [25] . By contrast, because of the retention of water by PAMPS [23] , no phase transition occurred in BG, which underwent a weak, gradual contraction with increasing C NaCl due to the screening of electrostatic repulsions within PAMPS and shrinkage of PNIPAm ( Supplementary Table S2 ). The normalized excess length of the BG stripes Δ f =( f BG − f PG )/ f PG , reached a maximum value at C NaCl =1.2 M ( Fig. 2a , inset). Figure 2: Variation in properties of the individual PG and BG components of the patterned gel sheet. ( a ) Relative change in the linear dimensions, f , of PG ( ○ ) and BG (□), plotted as a function of C NaCl . ( b ) Variation in the Young’s moduli of PG ( ○ ) and BG (□), plotted versus C NaCl . The error bars represent s.d. calculated from three measurements. Insets in a and b show the variation in the normalized difference in dimensions of PG and BG, Δ f , and the ratio of Young’s moduli, , respectively. Full size image Figure 2b shows the variation in the Young’s moduli, E PG and E BG , of PG and BG, respectively, plotted as a function of C NaCl . The value of E PG exhibited a twofold increase for 0.5≤ C NaCl ≤1.2 M (correlating with PNIPAm dehydration) and a further fivefold increase for 1.2≤ C NaCl ≤1.7 M (ascribed to the decrease in the configurational freedom of polymer chains, caused by the hydrated salt ions trapped in the collapsed gel) [26] . The value of E BG changed insignificantly, and the maximum in the ratio of Young’s moduli was achieved at C NaCl =1.7 M ( Fig. 2b , inset). Theoretical modelling We modelled the patterned gel sheet as a periodic structure of soft BG stripes and rigid PG stripes with initial widths and , respectively, and initial sheet thickness t 0 . In the NaCl solution, PG and BG stripes ( Fig. 3a ) shrink by different amounts. The acquired widths and thicknesses of the PG and BG stripes would be w PG , w BG , t PG and t BG , respectively, the ratio of their dimensions would be Δ f =( f BG − f PG )/ f PG ( Fig. 3a ), and the ratio of their Young’s moduli . Within an integrated sheet, the stripes are not free to keep their equilibrium length. Thus, any planar configuration of the sheet possesses a stretching energy. Similarly to narrow strips with an in-plane gradient in swelling [25] , [27] , a periodic gel sheet can reduce in-plane strain by buckling. Consider a configuration with a large-scale curvature 1/ R along the x -direction and a small-scale modulation of amplitude, η , along the y -direction ( Fig. 3b ). In such a configuration, the centerlines of the BG stripes form ‘rings’ with a radius R + η , compared with the radius R of the PG stripes ( Fig. 3d ). The BG stripes are, therefore, longer than the PG stripes. For given R and η , the length ratio of the stripes’ centre lines is Δ l =( l BG − l PG )/ l PG =( η / R ) and much of the stretching energy can be relaxed, if R and η are such that Δ l =Δ f . 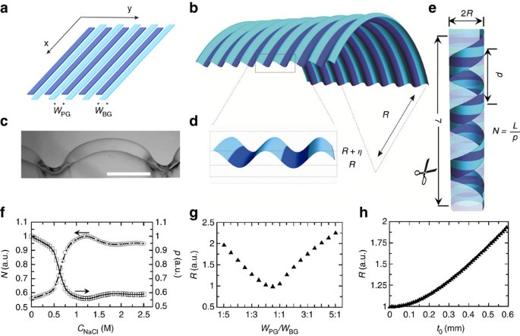Figure 3: Generation of helical structures with prescribed structural characteristics. (a) ‘Rest’ lengths of the stripes of PG and BG in the solution of NaCl. (b–d) Inward and outward buckling of the stripes of PG and BG, respectively, and the transformation of the shape of the gel sheet to accommodate the difference in lengths of the stripes. The image in (c) shows the cross-section of the surface of the helix formed in a 1-M solution of NaCl. Scale bar, 500 μm. (e) Generation of the helix with the radiusR, lengthL, number of turns,N, and pitchp. (f) Predicted variation inNandpwith increasingCNaCl. The values ofNandpwere calculated for the measured values of Δf(CNaCl) and(CNaCl) (presented inFig. 2a) forandt0/w0=0.25. (g) Predicted change inR, plotted as a function of the ratiowPG/wBG. The change inwPG/wBGwas achieved by increasingwPG(right arm) andwBG(left arm), while keeping the complementary stripe width constant. (h) Predicted variation inRversust0. Graphs in (g,h) were obtained for the values of Δfandmeasured atCNaCl=1.2 M. a.u. means arbitrary units. Figure 3: Generation of helical structures with prescribed structural characteristics. ( a ) ‘Rest’ lengths of the stripes of PG and BG in the solution of NaCl. ( b – d ) Inward and outward buckling of the stripes of PG and BG, respectively, and the transformation of the shape of the gel sheet to accommodate the difference in lengths of the stripes. The image in ( c ) shows the cross-section of the surface of the helix formed in a 1-M solution of NaCl. Scale bar, 500 μm. ( e ) Generation of the helix with the radius R , length L , number of turns, N , and pitch p . ( f ) Predicted variation in N and p with increasing C NaCl . The values of N and p were calculated for the measured values of Δf( C NaCl ) and ( C NaCl ) (presented in Fig. 2a ) for and t 0 / w 0 =0.25. ( g ) Predicted change in R , plotted as a function of the ratio w PG / w BG . The change in w PG / w BG was achieved by increasing w PG (right arm) and w BG (left arm), while keeping the complementary stripe width constant. ( h ) Predicted variation in R versus t 0 . Graphs in ( g , h ) were obtained for the values of Δ f and measured at C NaCl =1.2 M. a.u. means arbitrary units. Full size image To predict the dependence of sheet configuration on the modulated properties of the gel, we solved a simplified problem that involved several approximations (a more realistic model is included in Supplementary Discussion). As over most of the parameter range, we treated the PG as inextensible. Therefore, all the stretching energy is contained within the BG stripes, while the bending energy is contained within the PG stripes. In addition, we approximated the curvature in the y -direction as constant within each stripe ( Fig. 3c ). This approximation is satisfied in the experiments ( Fig. 3c ), and it is valid as long as the sheet thickness is not much smaller than the width of the stripes. Finally, based on the bending energy reduction arguments ( Supplementary Information ), we assumed that the curvatures in the x - and y -directions are comparable, thereby leading to . Under these approximations, the stretching and bending energies are , and , respectively. The resulting value of R is determined by the competition between these two contributions, that is, the stretching energy, which favours a buckled configuration with and the bending energy, which favours a flat configuration ( R →∞). Minimizing the energy yielded the selected value of R (see also Supplementary Discussion) In equation (1), the first ‘geometric’ term gives the value of R in an (approximate) stretch-free configuration (Δ f =Δ l ). It is independent of the sheet thickness and the Young’s moduli of the stripes and is dominant for thin sheets. The second, bending-driven term determines the deviation from the stretch-free configuration. This term favors sheet flattening (that is, the increase in R ), in order to reduce its bending energy, and it dominates at large sheet thicknesses and large ratios . In the experiments, the PG and BG stripes are oriented at an angle θ , which can be considered as an oblique cut from the cylindrical sheet [28] , that is, a helix ( Fig. 3e ). Together with the value of θ , equation (1) predicts all the trends in the variation of the structural characteristics of the helix. For example, the helix’s pitch p decreases with Δ f and increases with These competing effects occur simultaneously as C NaCl increases ( Fig. 2 ), leading to the initial decrease in p and increase in N , and their ‘saturation’ at high C NaCl ( Fig. 3f ), in qualitative agreement with experimental results ( Fig. 1c ). Other predictions of equation (1) include the variation in R with the ratio of widths of PG and BG stripes, w BG / w PG ( Fig. 3g ), and the increase in R with the thickness t 0 ( Fig. 3h ). The model does not provide the sign of bending curvature: the right- or left-handedness of the helix is equally possible, in agreement with experimental observations, as a result of the symmetry of the system along the z- (thickness) direction. In this respect, the proposed mechanism is intrinsically different from helix-forming mechanisms reported in earlier works. Validation of the theoretical model The predictive power of the model was validated by the ability to predict and generate new helical structures. First, we examined experimentally a non-monotonic variation in R versus ( Fig. 4a and Supplementary Fig. S8 ), which was in agreement with the results of modelling ( Fig. 3g ). Next, we used this effect to generate conical helixes. By incrementally reducing the ratio along the long axis of the gel sheet ( x axis), we formed a helix with a gradually increasing radius R ( Fig. 4b ). Moreover, by following guidance of Fig. 3h , we generated conical helices from the hydrogel sheet with the thickness gradually reducing along the x axis of the sheet (the width of the stripes of PG and BG was maintained constant) ( Fig. 4c ). 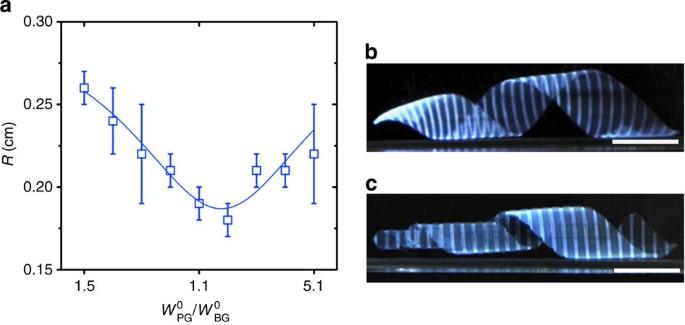Figure 4: Formation of conical helices. (a) Variation in the radius of the helix with the change inatCNaCl=1.2 M.t0=0.44 mm. The error bars represent s.d. values calculated from 10 measurements. (b) A conical helix generated in the NaCl solution by gradually increasing the value of(left to right) from 0.5 to 1.2 mm with a 0.025 mm increment per stripe at=1 mm (corresponding to the change in the ratiofrom 1:1.25 to 2:1).t0=0. 44 mm. (c) A conical helix formed in the NaCl solution by the gel sheet witht0changing (left to right) from 0.25 to 0.6 mm, at1 mm. In (b,c)CNaCl=1.0 M. Scale bar, 1 cm. Figure 4: Formation of conical helices. ( a ) Variation in the radius of the helix with the change in at C NaCl =1.2 M. t 0 =0.44 mm. The error bars represent s.d. values calculated from 10 measurements. ( b ) A conical helix generated in the NaCl solution by gradually increasing the value of (left to right) from 0.5 to 1.2 mm with a 0.025 mm increment per stripe at =1 mm (corresponding to the change in the ratio from 1:1.25 to 2:1). t 0 =0. 44 mm. ( c ) A conical helix formed in the NaCl solution by the gel sheet with t 0 changing (left to right) from 0.25 to 0.6 mm, at 1 mm. In ( b , c ) C NaCl =1.0 M. Scale bar, 1 cm. Full size image Multiple shape transformations Using the concept of small-scale modulation in properties of the material, we achieved discontinuous reversible transitions between the two stable helical shapes, each characterized by a different number of turns. We patterned the sheet with three types of periodic stripes in a sequence H 1 -H 2 -H 3 ( Fig. 5a ), corresponding to poly(hydroxyethylacrylamide- co - N -isopropylacrylamide)/PNIPAm (P(HEAm- co -NIPAm)/PNIPAm), P(HEAm- co -NIPAm), and P(HEAm- co -NIPAm)/PAMPS hydrogels, respectively. At 40 °C, above the dehydration temperature of P(HEAm- co -NIPAm)/PNIPAm of 34 °C, the stripes of H 1 shrank, and the regions of H 2 and H 3 remained soft and swollen. Under these conditions, a helix with N =1.9 was formed ( Fig. 5b ). Heating the system to 65 °C, above the dehydration temperature of P(HEAm- co -NIPAm) of 53 °C, led to the collapse of H 2 ( Supplementary Fig. S9 ), causing a sharp decrease in the dimensions of the swollen soft stripes (from H 2 +H 3 to H 3 ). In agreement with the prediction given in Fig. 3g , this effect resulted in an increase in the number of turns of the helix to N =2.5. 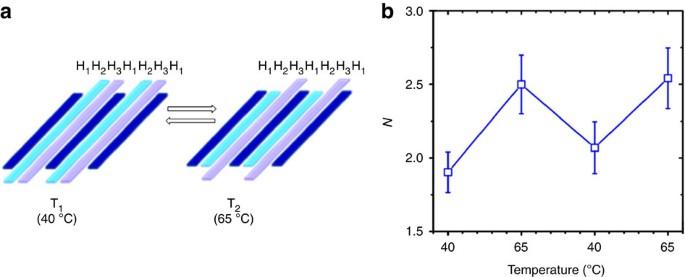Figure 5: Temperature-induced transitions between helical configurations. (a) Schematic of the temperature mediated change in dimensions of stripes of poly(hydroxyethylacrylamide-co-N-isopropylacrylamide)/PNIPAm (H1), P(HEAm-co-NIPAm) (H2) and P(HEAm-co-NIPAm)/PAMPS (H3) hydrogels. (b) Reversible discontinuous temperature-induced transitions between the two states of the helix with different number of turnsNin deionized water. The initial widths of the stripes in the as-prepared gel at 25 °C were 1.05 mm.t0=0.25 mm.θ=45°. The error bars denote s.d. values calculated from five measurements. Figure 5: Temperature-induced transitions between helical configurations. ( a ) Schematic of the temperature mediated change in dimensions of stripes of poly(hydroxyethylacrylamide- co - N -isopropylacrylamide)/PNIPAm (H 1 ), P(HEAm- co -NIPAm) (H 2 ) and P(HEAm- co -NIPAm)/PAMPS (H 3 ) hydrogels. ( b ) Reversible discontinuous temperature-induced transitions between the two states of the helix with different number of turns N in deionized water. The initial widths of the stripes in the as-prepared gel at 25 °C were 1.05 mm. t 0 =0.25 mm. θ =45°. The error bars denote s.d. values calculated from five measurements. Full size image The reported shaping mechanism enabled ‘programming’ of multiple 3D shape transformations, beyond the generation of helical structures, thereby making the material reconfigurable and adaptable to ambient conditions. We demonstrated this unique feature by designing a gel sheet composed of stripes of poly(acrylamide- co -butyl methacrylate) gel (H 1 ), poly( N -vinyl imidazole)/poly(acrylamide- co -butyl methacrylate) (H 2 ) and poly(acrylamide- co -butyl methacrylate)/poly(methacrylic acid) (H 3 ). The stripes of H 2 and H 3 were running at θ of 0 and 45°, respectively, to the long axis of the gel sheet, as shown in Fig. 6a . Under close-to-neutral conditions (pH=6.8), the cationic and anionic stripes were not activated and the sheet acquired a planar configuration ( Fig. 6a′ ). The pH-responsive regions of the gel selectively swelled under acidic and basic conditions ( Fig. 6b ). At pH=2.3, the cationic H 2 stripes containing poly( N -vinyl imidazole) expanded, leading to a planar-to-arc transition of the sheet ( Fig. 6b′ ). At pH=9.5, the anionic stripes containing poly(methacrylic acid) swelled, causing a planar-to-helical shape transformation ( Fig. 6c′ ). 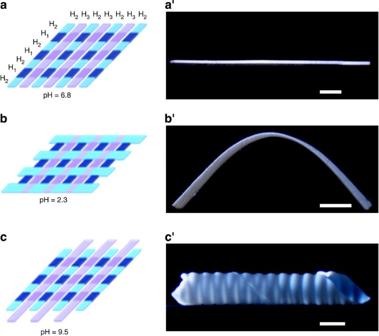Figure 6: Multiple shape transformations programmed in the gel sheet. Schematic of the sheet composed of stripes of poly(acrylamide-co-butyl methacrylate) gel (H1), poly(N-vinyl imidazole)/poly(acrylamide-co-butyl methacrylate) (H2) and poly(acrylamide-co-butyl methacrylate)/poly(methacrylic acid) (H3) at pH=6.8. The regions of H1, H2and H3are shown with dark-blue, light-blue and purple colours, respectively. (a′) A planar gel sheet patterned as shown inaat pH=6.8. (b) Schematic of the gel sheet patterned as shown in (a) and exposed to acidic solution at pH=2.3. (b′) An arc-shape gel sheet as in (b) at pH=2.3. (c) Schematic of the gel patterned as shown in (a) and exposed to basic solution at pH=9.5. (c′) A helix formed by the gel sheet shown in (c) at pH=9.5.1 mm,t0=0.44 mm. The stripes of H2and H3are running atθ=0 andθ=45°, respectively, to the long axis of the gel sheet. Figure 6: Multiple shape transformations programmed in the gel sheet. Schematic of the sheet composed of stripes of poly(acrylamide- co -butyl methacrylate) gel (H 1 ), poly( N -vinyl imidazole)/poly(acrylamide- co -butyl methacrylate) (H 2 ) and poly(acrylamide- co -butyl methacrylate)/poly(methacrylic acid) (H 3 ) at pH=6.8. The regions of H 1 , H 2 and H 3 are shown with dark-blue, light-blue and purple colours, respectively. ( a′ ) A planar gel sheet patterned as shown in a at pH=6.8. ( b ) Schematic of the gel sheet patterned as shown in ( a ) and exposed to acidic solution at pH=2.3. ( b′ ) An arc-shape gel sheet as in ( b ) at pH=2.3. ( c ) Schematic of the gel patterned as shown in ( a ) and exposed to basic solution at pH=9.5. ( c′ ) A helix formed by the gel sheet shown in ( c ) at pH=9.5. 1 mm, t 0 =0.44 mm. The stripes of H 2 and H 3 are running at θ =0 and θ =45°, respectively, to the long axis of the gel sheet. Full size image This study offers a new ‘small-scale’ strategy for the fabrication of self-shaping materials and the design of stimuli-responsive fibrous-like composite materials. By using advances in polymer patterning [29] , the length scale of the modulation in the properties of gel sheets can be reduced to micro- or nanometre range, leading to the miniaturization of the resulting self-shaped structures. The integration of multiple, hierarchical, small-scale structural components in planar sheets paves the way for multiple shape transformations of planar sheets, with distinct material shapes under selected ambient conditions. The approach can be extended to elastomers, liquid crystalline polymers, electroactive polymers and hybrid polymer-inorganic materials, thereby introducing functionality into shape transitions. Another important implication of the proposed chemo-mechanical system is its relevance for the current understanding of the deformation and actuation of fibrous living tissues [15] . Furthermore, the proposed theoretical model explains the principle that governs the development of curvature in thin gel sheets, in particular, for helixes, via a mechanism that is qualitatively different from any formerly studied helix-forming mechanism. The model provides an analytical expression, which links the local properties of the structural components of the gel sheet to the global (macroscopic) structural characteristics of the helix, and provides guidance for the design of new gel shapes. Photopatterning A PG with dimensions of 75 × 50 × 0.44 mm (length × width × thickness) was synthesized by photoinitiated polymerization of NIPAm, MBAA and a photoinitiator 2,2'-azo- bis -(2-methylpropionamidine) (V-50) in an aqueous solution. The reaction mixture was introduced into the reaction cell comprising two 1 mm-thick glass slides separated with a 0.5 mm-thick silicone rubber spacer. The cell was exposed for 25 s to ultraviolet light irradiation (365 nm, Hönle, UV Print at intensity 9 mW/cm 2 ). The PNIPAm gel was incubated for 1 day in deionized water and subsequently, swollen for 2 days with an aqueous solution of AMPS, MBAA and V-50. The swollen gel sheet was transferred into the reaction cell and a mask was placed above the top glass slide. Unless specified, the mask was prepared by ink-jet printing of 1-mm-wide black stripes separated from each other by 1 mm-wide spacing. The angle between the stripes and the long axis of the mask varied from −45 to 90°. The swollen gel was exposed for 70 s to the ultraviolet light irradiation. To avoid thermally induced phase transition of PNIPAm [21] , polymer synthesis was carried out in a reaction cell placed on a bed of ice. The recipes used for the first-step and the second-step synthesis are shown in Supplementary Table S3 . Following the second polymerization step, a BG with an interpenetrating network structure formed in the light-exposed regions from PAMPS and PNIPAm. The top glass slide of the polymerization cell was removed, the patterned gel sheet was cut into rectangular samples with dimensions 65 × 10 × 0.44 mm, detached from the bottom glass slide and immersed into the solution of NaCl or deionized water at 45 °C. Following 2–3 h incubation, the unreacted monomer and free (non-crosslinked) polymer molecules diffused from the light-protected regions, while the aqueous medium diffused into the gel, and the planar sheet transformed into a helix. For optional control of helix chirality, after the second polymerization step, the sheet was exposed to the ambient air for 5–8 min. The surface of the patterned gel exposed to the ambient atmosphere formed the inner surface of the helix, thereby determining the handedness of the helix. The individual non-patterned PG and BG samples were polymerized using a similar two-step procedure without a mask. The polymer content in the as-prepared PG and BG samples was determined after drying the gels in a vacuum oven at 60 °C for 10 h. The polymer contents in PG and BG regions of the hydrogel sheets were 16.0 wt% and 28.2 wt%, respectively. The mass ratio between PNIPAm and PAMPS in BG was 4:3. Variation in the ratio of volumes of the gels in solutions with varying C NaCl The ratio of volumes of the binary to PGs was determined as V BG / V PG =( f BG / f PG ) [3] , where f BG and f PG are the relative changes in linear dimensions of BG and PG disks (defined in the main.text). Measurements of the Young’s moduli of the gels Experiments were conducted for 0.44 mm-thick PG and BG disks using the Instron 5848 Micro-Tester. Samples with a diameter of 13.2 mm were immersed overnight in solutions of NaCl at 0≤ C NaCl ≤2.5 M at 23 °C. The thickness of the samples varied with the C NaCl and was taken into account in the measurements of Young’s moduli. Compression tests were carried out with a velocity of compression of 0.1 mm min −1 . The values of Young’s moduli were calculated from the slopes of the stress–strain curves with strain below 10%. Other experimental details are described in Supplementary Methods . How to cite this article: Wu, Z. L. et al. Three-dimensional shape transformations of hydrogel sheets induced by small-scale modulation of internal stresses. Nat. Commun. 4:1586 doi: 10.1038/ncomms2549 (2013).